Benzene construction via organocatalytic formal [3+3] cycloaddition reaction The benzene unit, in its substituted forms, is a most common scaffold in natural products, bioactive molecules and polymer materials. Nearly 80% of the 200 best selling small molecule drugs contain at least one benzene moiety. Not surprisingly, the synthesis of substituted benzenes receives constant attentions. At present, the dominant methods use pre-existing benzene framework to install substituents by using conventional functional group manipulations or transition metal-catalyzed carbon-hydrogen bond activations. These otherwise impressive approaches require multiple synthetic steps and are ineffective from both economic and environmental perspectives. Here we report an efficient method for the synthesis of substituted benzene molecules. Instead of relying on pre-existing aromatic rings, here we construct the benzene core through a carbene-catalyzed formal [3+3] reaction. Given the simplicity and high efficiency, we expect this strategy to be of wide use especially for large scale preparation of biomedicals and functional materials. Multi-substituted benzenes are widely present in natural products. In industry, these benzene frameworks are nearly unavoidable in preparing most of today’s biomedicals, fine chemicals and polymer materials. The functions of the benzene-containing molecules are determined by the identity and substitution patterns of the substituents installed on the benzene unit. Exemplified in Fig. 1a are one natural product (salvadorin) [1] and two synthetic bioactive molecules [2] , [3] containing a benzene core bearing four substituents. Most synthetic methods in synthesizing such multi-substituted aromatics start with pre-existing benzene unit by replacing hydrogen with other functional groups. The classic approach relies on stepwise electrophilic substitution (such as Friedel–Crafts reaction) or electrophilic halogenation and successive transition metal-catalyzed couplings. However, regio-selectivity and chemo-selectivity normally require rather tedious functional group (including protecting group) manipulations. For example, the classic synthesis of a 2,4,6-trisubstituted benzoate needs the introduction of a temporary amine group to ensure selectivities in a key bromination reaction step [4] , and the overall synthesis requires over eight steps ( Fig. 1b ). Another approach for access to substituted benzenes is based on transition metal-catalyzed direct C–H activations [5] , [6] , [7] , [8] . While providing impressive shortcuts for benzene substitutions, this C–H activation method has its own limitations. For example, the presence of directing groups (for coordination with the metal catalyst) is often necessary and the instruction of multiple substituents is difficult (in part due to steric congestion). In a different direction for substituted benzene synthesis, the benzene core is newly formed. Representative methods include transition metal-catalyzed [2+2+2] or [4+2] reactions such as acetylene trimerizations developed by Reppe et al. [9] , [10] , [11] In this cycloaddition approach, partial or complete intramolecular reaction is usually indispensable to ensure the regio-selectivity. 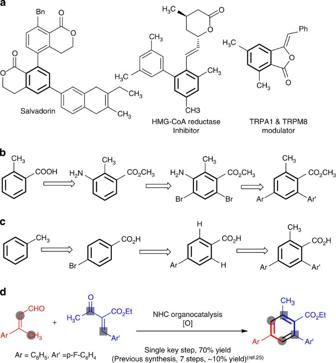Figure 1: Multi-substituted benzenes and their synthesis. (a) examples of natural products and bioactive synthetic compounds containing multi-substituted benzene. (b) it took about eight steps for the classical substitution methods to synthesize a 2,4,6-trisubstituted benzoate. (c) transition metal-catalyzed C–H activation methods provides a shortcut (about five steps) for the synthesis. (d) this work: single key step reaction to afford tetra-substituted benzenes via organocatalyzed formal [3+3] cycloaddtion. Figure 1: Multi-substituted benzenes and their synthesis. ( a ) examples of natural products and bioactive synthetic compounds containing multi-substituted benzene. ( b ) it took about eight steps for the classical substitution methods to synthesize a 2,4,6-trisubstituted benzoate. ( c ) transition metal-catalyzed C–H activation methods provides a shortcut (about five steps) for the synthesis. ( d ) this work: single key step reaction to afford tetra-substituted benzenes via organocatalyzed formal [3+3] cycloaddtion. Full size image Here we report a new strategy for highly effective access to multi-substituted benzenes through the construction of the benzene core via a formal [3+3] cycloaddition reaction ( Fig. 1d ). Our approach uses enals readily prepared in three steps and unsaturated ketones as the starting material and N-heterocyclic carbene (NHC) as the organic catalyst [12] , [13] , [14] , [15] , [16] , [17] , [18] , [19] , [20] , [21] , [22] , [23] , [24] . It is a single-step reaction that affords tetra-substituted benzenes (2,4,6-trisubstituted benzoate and its analogues) with high yield. In comparison, previous approaches to this class of molecules typically need seven steps with less than 10% overall yields [25] ( Fig. 1d ). A plausible pathway of our NHC-catalyzed [3+3] cycloaddition reaction involving formal α-, and γ-carbon activations of enal is illustrated in Fig. 2 . Briefly, addition of the carbene catalyst to the aldehyde moiety of enal followed by deprotonation forms Breslow intermediate I [26] , [27] , [28] . This process is followed by oxidative transformation [29] , [30] , [31] , [32] , [33] , and former enal γ-CH deprotonation [33] leads to vinyl enolate intermediate III . Notably, similar vinyl enolate intermediate could also be accessed from ketenes [34] by Ye or esters in our laboratory [35] . Nucleophilic Michael-type addition of the γ-carbon of III to enone 2 affords intermediate IV bearing a NHC-bound α,β-unsaturated ester moiety. Subsequent γ-CH deprotonation of IV lead to dienolate intermediate V that undergoes an intramolecular aldol to form a cyclic intermediate VI . Intramolecular ester formation with the release of NHC catalyst yields a bicyclic adduct VII containing a four-membered β-lactone. Spontaneous decarboxylation [36] , [37] , [38] , [39] and oxidation [40] , [41] , [42] of VII effectively affords benzene product bearing four substituents in predictable substitution patterns. Decarboxylation of β-lactone fused with a six-membered ring similar to intermediate VII is a highly effective process, as exemplified in Lupton’s [4+2] reaction via carbene catalysis [39] . 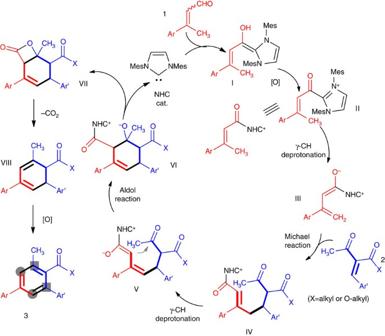Figure 2: Postulated pathway. Addition of carbene catalyst to aldehyde followed by oxidative transformation and γ-CH deprotonation leads to intermediateIII, which undergoes Michael addition to2and gives intermediateIV. Subsequent γ-CH deprotonation ofIVlead toV, after intramolecular adol reaction, decarboxylation and oxidation, finally gives a benzene product bearing four substituents in predictable substitution patterns. Mes, 2,4,6-trimethylphenyl. Cat., catalyst. Figure 2: Postulated pathway. Addition of carbene catalyst to aldehyde followed by oxidative transformation and γ-CH deprotonation leads to intermediate III , which undergoes Michael addition to 2 and gives intermediate IV . Subsequent γ-CH deprotonation of IV lead to V , after intramolecular adol reaction, decarboxylation and oxidation, finally gives a benzene product bearing four substituents in predictable substitution patterns. Mes, 2,4,6-trimethylphenyl. Cat., catalyst. Full size image Reaction optimization We started by using enal 1a and enone 2a as the model substrates, in the presence of 2 equiv. quinone 4 as an oxidant [29] , [30] , [31] , [32] , [33] and Cs 2 CO 3 as a base. No formation of the proposed benzene 3a was observed in the absence of an NHC precatalyst ( Table 1 , entry 1). The N -methyl imidazolium NHC A (ref. 43 ) and N -phenyl imidazolium B could not initiate the reaction ( Table 1 , entries 2–3). We then found that with N -Mes imidazolium C (ref. 44 ) as the NHC precatalyst, the proposed product 3 was formed in 88% isolated yield ( Table 1 , entry 4). Triazolium-based NHCs behaved similarly as the imidazolium catalysts: triazolium D (ref. 45 ) (with a N -phenyl substituent) could not catalyze the reaction; while the use of triazolium E (ref. 46 ) with a N -mesityl substituent could lead the formation of 3 in 47% yield ( Table 1 , entries 5–6). Thiazolium-based NHCs F (ref. 47 ) or G (ref. 48 ) could not initiate the reaction ( Table 1 , entries 7–8). We then evaluated the effects of solvents and bases. Although the combination of tetrahydrofuran and Cs 2 CO 3 was optimal, other common organic solvents (such as CH 2 Cl 2 , toluene, CH 3 CN and DMF) and organic/inorganic bases (such as Et 3 N, DBU, t BuOK and K 2 CO 3 ) could also be used (see the Supplementary Table 1 ). Further investigation showed that the catalyst loading of C could be decreased to 5 mol% with acceptable 76% yield ( Table 1 , entry 9). Table 1 Condition optimization for NHC-catalyzed [3+3] benzene construction. Full size table Scope of enal substrates With an acceptable reaction condition in hand ( Table 1 , entry 9), the scope of the reaction was evaluated. To demonstrate broader synthetic utility of this method, we chose enone 2b bearing an alkene group (amenable for further transformation) as a model enone substrate to study the generality of the enal substrates ( Fig. 3 , products 3b – j ). Both electron-donating (products 3c – d , 3f ) and electron-withdrawing group (products 3e , 3g ) at the p- position (products 3c – e ) or m- position (products 3f – g ) of the β-phenyl group were well-tolerated. Replacement of the β-phenyl substituent with a naphthyl (product 3h ) or heteroaryl unit (products 3i – j ) had little effect on the reaction outcome. It is worth to note that E- or Z- isomer of enal 1 gave essentially the same yields, so a mixture of E- / Z- enals can be directly used. 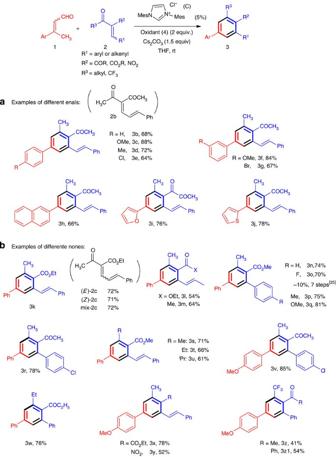Figure 3: Substrate scope. (a) Examples of different enals: study of enal substrate generality with ketone2bas a model enone substrate. (b) Examples of different enones: study of enones scope with aldehydes1a(Ar=C6H5) and1b(Ar=4-OCH3-C6H4) as model nucleophile. Ph, phenyl; Me, methyl; Et, ethyl. Figure 3: Substrate scope. ( a ) Examples of different enals: study of enal substrate generality with ketone 2b as a model enone substrate. ( b ) Examples of different enones: study of enones scope with aldehydes 1a (Ar=C 6 H 5 ) and 1b (Ar=4-OCH 3 -C 6 H 4 ) as model nucleophile. Ph, phenyl; Me, methyl; Et, ethyl. Full size image Scope of enone substrates With aldehydes 1a and 1b (Ar=4-OCH 3 -C 6 H 4 ) as model nucleophile, the scope of enones was also examined. As shown in Fig. 3 (products 3k – z1 ), in nearly all cases, the reaction proceeded smoothly at room temperature to give polysubstituted benzenes in moderate to good yields. Notably, the E -/ Z -configuration of enone 2 did not affect the reaction outcomes either (for example, see product 3k ), which greatly simplify substrate preparation process. Both electron-rich (products 3p – q ) or electron-deficient (products 3o and 3r ) aromatic groups, as well as vinyl groups (products 3k – m ) were all tolerated in the β-substituent (R 2 ) of the enone substrates. α-Substituent (R 3 ) of the enone substrates can be electron-deficient units such as acyl( 3m , 3r , 3v – 3w ), ester ( 3k – 3l , 3n–q ) or nitro ( 3y ) groups. Substituent in the carbonyl group of enones 2 (R 4 ) can be a different alkyl group including methyl ( 3k – q , 3r – s ), ethyl ( 3t and 3w ), isopropyl ( 3u ) or trifluoromethyl ( 3z – z1 ) group. It is important to note that these polysubsituted benzene molecules were difficult to prepare previously. For example, previous method for the synthesis of benzoate 3o required seven steps with less than 10% overall yields [25] ; previous synthesis of 3p and 3q needed a three-step reaction with 35 and 39% overall yield [49] , respectively. Our method also provides effective access to aromatic molecules with trifluoromethyl (CF 3 ) substituent. In organic synthesis, regioselective C–H trifluoromethylation [50] , [51] or methylation [52] , [53] , [54] of aryl molecules still remains challenging despite the rapid development in recent years. Product transformation We next demonstrated effective transformation of our catalytic reaction products to bicyclic and multicylic aromatic molecules that are found as a key scaffold in natural products and functional synthetic molecules. For example, the multisubsituted benzene adduct 3b could be transformed to indene 7 (ref. 55 ) via reduction followed by Lewis acid-mediated cyclization; 2,4,6-trisubstituted benzoate 3n can be transformed to fluorenone 5 (refs 56 , 49 ) or isoindolone 6 (ref. 57 ) via straightforward processes ( Fig. 4 ). 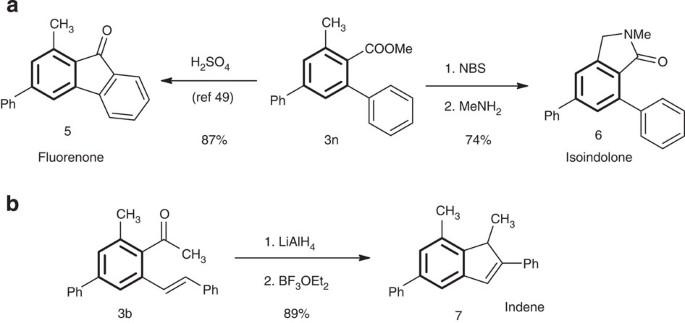Figure 4: Synthetic applicability. (a)3ncan be transfomed to fluorenone5or isoindolone6via straightforward processes. (b)3bcould be transformed to indene7via reduction followed by Lewis acid-mediated cyclization. NBS,N-bromosuccinimide. Figure 4: Synthetic applicability. ( a ) 3n can be transfomed to fluorenone 5 or isoindolone 6 via straightforward processes. ( b ) 3b could be transformed to indene 7 via reduction followed by Lewis acid-mediated cyclization. NBS, N -bromosuccinimide. Full size image In summary, we have developed a NHC organocatalytic strategy for the formal [3+3] construction of multi-substituted benzenes. Our method directly employs commercially available or easily accessible enals and enones to construct benzene framework with excellent regioselectivities, offering useful insights into the design of concise synthetic strategies for complex molecules. Further studies regarding reaction mechanisms, synthetic applications and axial chirality controls (for the formation of substituted benzene products) are under progress in our laboratory. Materials For 1 H, 13 C and 19 F NMR spectra of compounds in this manuscript, see Supplementary Figs 1–32 . For details of the synthetic procedures, see Supplementary Methods . Synthesis of 3 Under N 2 atmosphere, a solution of enal (0.1 mmol), enone (0.1 mmol), oxidant 4 (82 mg, 0.2 mmol), Cs 2 CO 3 (48.7 mmg, 0.15 mmol) and imidazolium C (1.7 mg, 0.005 mmol) in 1.0 ml tetrahydrofuran was stirred at room temperature for 8 h. The mixture was concentrated under reduced pressure and purified by silica gel column chromatography to afford the corresponding product 3 . How to cite this article: Zhu, T. et al. Benzene construction via organocatalytic formal [3+3] cycloaddition reaction. Nat. Commun. 5:5027 doi: 10.1038/ncomms6027 (2014).